Catalytic subsurface etching of nanoscale channels in graphite Catalytic hydrogenation of graphite has recently attracted renewed attention as a route for nanopatterning of graphene and to produce graphene nanoribbons. These reports show that metallic nanoparticles etch the surface layers of graphite or graphene anisotropically along the crystallographic zig-zag ‹11–20› or armchair ‹10–10› directions. The etching direction can be influenced by external magnetic fields or the supporting substrate. Here we report the subsurface etching of highly oriented pyrolytic graphite by Ni nanoparticles, to form a network of tunnels, as seen by scanning electron microscopy and scanning tunnelling microscopy. In this new nanoporous form of graphite, the top layers bend inward on top of the tunnels, whereas their local density of states remains fundamentally unchanged. Engineered nanoporous tunnel networks in graphite allow for further chemical modification and may find applications in various fields and in fundamental science research. Local hydrogenation of graphite catalysed by metallic nanoparticles has been known since the 1970s (refs 1 , 2 , 3 ). This process results in straight nanoscale channels that have intersecting angles of integer multiples of 30° (ref. 2 ). In recent years it has attracted renewed attention as a possible route for nanopatterning of graphene, especially for the production of graphene nanoribbons. Metallic nanoparticles etch the surface layers of graphite [1] , [2] , [3] , [4] , [5] , [6] , [7] , [8] , as well as single-layer graphene sheets [9] , [10] . The process is anisotropic along the crystallographic high-symmetry directions, that is, the zigzag ‹11–20› or armchair ‹10–10› directions. Nanoparticles consisting of various metals, such as Ni [2] , [8] , [9] , [10] , Fe [2] , [7] , Pt [3] , Co [2] , [4] , [5] and Ag [6] , are known to etch channels on graphite surfaces. It was shown that the etching direction could be influenced by an external magnetic field when Co particles were used [11] . Similarly, the etching direction on mono and few-layer graphene could be controlled by the structure of the substrate [12] , [13] . To date, clear evidence has been reported only for open channels on the surface of graphite, whereas subsurface etching remains unclear [4] , [5] , [8] . In this study, we demonstrate the subsurface etching of highly oriented pyrolytic graphite (HOPG) by Ni nanoparticles. Besides the well-known open channels, a network of tunnels is produced, which can be probed by scanning electron microscopy (SEM) and scanning tunnelling microscopy (STM). By semiempirical quantum chemical and density functional theory calculations, we are able to show that the top layers bend inward on top of the tunnels, whereas their local density of states remains fundamentally unchanged. The etched material presents a new nanoporous form of graphite with high potential for applications. Sample preparation In this work, HOPG was etched by the two-step procedure described previously [9] . A controlled oxidation step creates etch pits in the surface that expose the edges of graphene sheets as nucleation sites. Subsequently deposited Ni nanoparticles resting at these artificial and at the natural step edges serve as catalyst for hydrogenation of carbon when the sample is exposed to high temperature in H atmosphere (see Methods for more details). It is understood that the nanoparticle is dragged into the void where carbon atoms have been removed at the edge of the sheet, catalyses further hydrogenation of carbon and successively etches a channel from the edge into the sheet, following the main symmetry directions of carbon lattice [1] , [3] , [5] , [6] , [7] , [8] , [9] , [10] (see also Fig. 1a ). The width of the channels is correlated to the particles’ size, which was polydisperse in our preparation method. 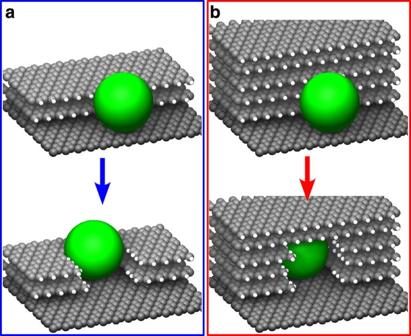Figure 1: Schematic image of the channel formation. Etching starts at natural or artificial step edges of the graphite layers. The carbon is drawn as grey sphere, a sheet termination by hydrogen is drawn as white sphere. The metallic particle is symbolized by a green ball for simplicity. A particle that is in contact with the side termination of the carbon sheets of the edge (a,b, upper panel) catalyses carbon hydrogenation. It is drawn into the void where it catalyses further hydrogenation, etching a channel into the carbon layers (a,b, lower panel). The dimensions of the channel are determined by the size of the particle. Particles with a diameter larger than the step edge etch open trenches (a), whereas a particle smaller than the step edge can etch a tunnel (b). Figure 1: Schematic image of the channel formation. Etching starts at natural or artificial step edges of the graphite layers. The carbon is drawn as grey sphere, a sheet termination by hydrogen is drawn as white sphere. The metallic particle is symbolized by a green ball for simplicity. A particle that is in contact with the side termination of the carbon sheets of the edge ( a , b , upper panel) catalyses carbon hydrogenation. It is drawn into the void where it catalyses further hydrogenation, etching a channel into the carbon layers ( a , b , lower panel). The dimensions of the channel are determined by the size of the particle. Particles with a diameter larger than the step edge etch open trenches ( a ), whereas a particle smaller than the step edge can etch a tunnel ( b ). Full size image SEM and STM investigations The SEM image of such a sample shows indeed etch channels of different width that are mainly oriented along a few preferred directions ( Fig. 2a ). On closer inspection, two different types of channels can be distinguished: The first type (one is marked by a blue arrow in Fig. 2a ) appears brighter directly at the edge. The other type (red arrow) does not show this effect. This difference is best seen in the intensity profile ( Fig. 2b ) along the white line in Fig. 2a . In SEM imaging, it is a well-known phenomenon that edges within the scattering cloud of the electron beam give a higher secondary electron (SE) yield and appear brighter than plain surface parts [14] . Hence, channels with bright edges indicate open channels (trenches). The missing of enhanced SE emission in the second type of channels is not dependent on the channel width. It, therefore, cannot be assigned to resolution limits of the apparatus, but implies a different channel morphology. 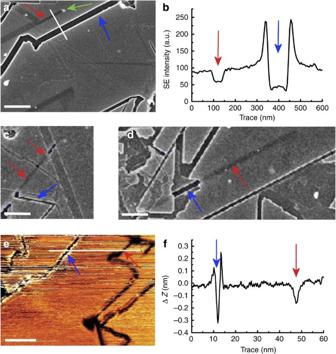Figure 2: Appearance of etch channels in SEM and STM images. SEM (a,c,d) and STM images (e) show open channels (blue arrows), closed channels (red arrows) and subsurface catalyst particles (green arrow). An averaged SE intensity profile (b) and an apparent height profile (f) along the white lines inaandehighlight the different contrast of trenches and tunnels. Switching between trench and tunnel contrast along channels is found, where covering layers are partially removed (c,d). Scale bars, 500 nm (a,c,d), 20 nm (e). STM image in constant current mode:U=−1 V,I=0.28 nA. Figure 2: Appearance of etch channels in SEM and STM images. SEM ( a , c , d ) and STM images ( e ) show open channels (blue arrows), closed channels (red arrows) and subsurface catalyst particles (green arrow). An averaged SE intensity profile ( b ) and an apparent height profile ( f ) along the white lines in a and e highlight the different contrast of trenches and tunnels. Switching between trench and tunnel contrast along channels is found, where covering layers are partially removed ( c , d ). Scale bars, 500 nm ( a , c , d ), 20 nm ( e ). STM image in constant current mode: U =−1 V, I =0.28 nA. Full size image In STM investigations of the same sample, we also observe two different channel types ( Fig. 2e ). The height profile ( Fig. 2f ) along the white trace in Fig. 2e illustrates the differences. Some channels, marked by blue arrow, are imaged in the same way as step edges of HOPG. The apparent height Δ z shows an enhancement near a step edge of a monolayer (ML) or multiple ML height. The enhancement is always found on the upper terrace and is due to an altered electronic structure [15] , [16] , [17] , [18] , [19] , [20] , [21] or backfolding of the sheet [15] , [22] , [23] near the edge. This channel corresponds to a trench where the top layers of graphite have been etched away by an Ni particle. A second type of channel (red arrow in Fig. 2e ) does not show this edge enhancement and was investigated in detail. We find no reconstruction of graphite or height-enhancement near the step edge for the channel in Fig. 3a , as is clearly seen in the height profiles along the traces 1, 2, which are plotted in Fig. 3b . Furthermore, the channel-depth with 45–50 pm is by far too small for an ML step on graphite (Δ z =350 pm). 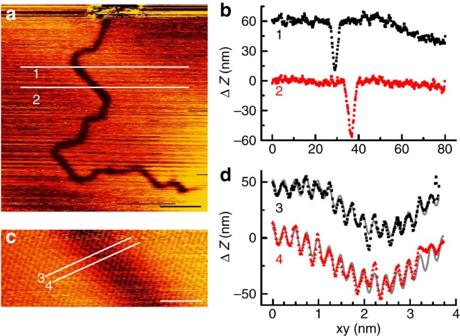Figure 3: High-resolution STM images and height profiles of a tunnel. The height profiles (b) of the traces marked 1, 2 in the STM image (a) show a smooth sub-monolayer depression without edge enhancement. The atomically resolved STM image of the same area (c) shows an intact top graphene sheet. The height profiles (d) along the traces 3, 4 incshow unperturbed periodicity when fitted with a sine function. Black and red symbols: measured height from STM, grey line: sine function superimposed onto third order polynomial (flexed beam model). Scale bars, (a) 20 nm, (b) 2 nm, all images constant current mode,U=0.7 V,I=0.98 nA (a),I=0.74 nA (b). Figure 3c shows the same region with atomic resolution. It is obvious that the periodic structure of the top graphene layer is unperturbed throughout the channel’s area. The height profiles along traces 3, 4 ( Fig. 3d ) can be fitted by a cosine function of periodicity 0.247 nm superimposed onto a third-grade polynomial (describing a flexed beam). We, therefore, conclude that the surface sheet of graphite is intact, but appears to be sagged down along a trace of similar orientation and width as an etch trench. All sagged traces of this kind have a connection to etch pits, step edges or other etch trenches. In Fig. 3a , this is seen at the top of the image. We thus conclude that the etching process is not limited to the surface, but also takes place in the material below the surface: Whenever the catalytic particle’s diameter is smaller than the height of the edge, it can start to etch a tunnel, leaving the upper sheets intact ( Fig. 1b ). Figure 3: High-resolution STM images and height profiles of a tunnel. The height profiles ( b ) of the traces marked 1, 2 in the STM image ( a ) show a smooth sub-monolayer depression without edge enhancement. The atomically resolved STM image of the same area ( c ) shows an intact top graphene sheet. The height profiles ( d ) along the traces 3, 4 in c show unperturbed periodicity when fitted with a sine function. Black and red symbols: measured height from STM, grey line: sine function superimposed onto third order polynomial (flexed beam model). Scale bars, ( a ) 20 nm, ( b ) 2 nm, all images constant current mode, U =0.7 V, I =0.98 nA ( a ), I =0.74 nA ( b ). Full size image It might be argued that a very blunt tip would not resolve the depth and the abrupt height change of a narrow ML trench. However, at a ML step edge, the atomic positions change laterally by 71 pm, and the positions described by the maxima of the sine are shifted by half a period. Although the lateral shift might be difficult to recognize, the π -shift in the sine is clearly missing. For a deeper trench with the maxima in phase, again the atomic resolution becomes impossible with the tip more than an ML further away from the surface. The perfect fit of the sine function beside and on the channel indicates that the top sheet is intact and that the tunnel is covered by at least two layers of graphene (see Supplementary Methods for imaging details). The apparent sagging above the tunnel is not necessarily due to sample topography as will be discussed below. The existence of etch trenches and tunnels explains the findings in the SEM images ( Fig. 2a ) straight away. The contrast enhancement due to increased SE emission from the edge of a trench (blue arrows) cannot occur for a tunnel’s edge buried inside the bulk material (red arrows). Reduced SE generation in the tunnel (no material to scatter) accounts for the effect that tunnels appear darker than the surroundings. The differences can be seen very clearly in Fig.2c where the material above a tunnel is partially removed. In contrast, the interpretation of the STM images of tunnels is not straightforward, because the tunnelling current depends on the tip-sample distance, as well as on the local density of states of the sample. Therefore, the apparent sagging of the graphene layers covering the tunnels as observed in STM may have different causes: (i) graphene layers covering the tunnel may form a sagging ceiling, or (ii) the density of states is decreasing towards the centre-line of the tunnel, or (iii) a mixture of both effects. Modelling of the tunnels To gain better understanding of these phenomena, we performed semiempirical quantum chemical calculations using the modified neglect of diatomic differential overlap method [24] . We modelled the tunnel as a stack of several graphene sheets, periodic in the zigzag ‹11–20› and armchair ‹10–10› directions, in which a tunnel running along ‹10–10› was created in the centre (see Methods and Supplementary Fig. S1 for details of the stacking geometry). The sidewall of the tunnel corresponds to a straight armchair edge and was saturated with hydrogen atoms. The tunnel geometry was varied having different width and one, two, or three covering layers. For these models, we performed an energy minimization, permitting all atoms to follow their local gradient until equilibrium was reached. Some of the relaxed structures of lowest energy are shown in Fig. 4a–d (for all structures see Supplementary Table S1 ). For all models, a downward bending of the top layers was observed. For tunnels of the same width ( Fig. 4a–c ), the deflection Δ z of the topmost carbon sheet out of its bulk position decreases from 180 pm for one cover layer to 51 pm for three cover layers. For a single cover layer, we observed much stronger bending for the wider tunnel, Δ z =280 pm ( Fig. 4d ). 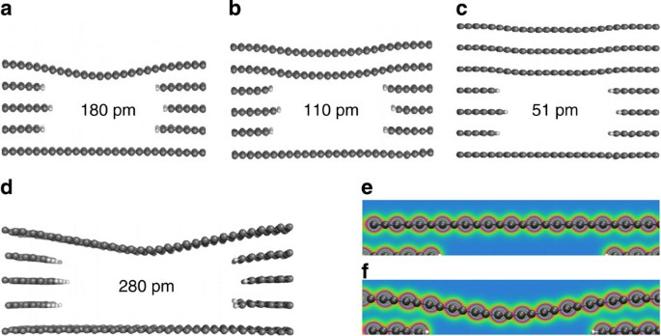Figure 4: Relaxed lowest-energy structures and electron density of tunnels. Structuresa–dare the lowest-energy structures after the relaxation. In all lowest-energy structures, the top sheet bends downward. The numbers give the maximum deviation Δzof the topmost layer from the straight configuration. The bending of surface sheets decreases with increasing number of covering layers (a–c) and increases with tunnel width (a,d). In density functional theory calculations, no reconfiguration of the electron density is found due to the missing of layers underneath the top sheet (e) nor due to bending (f). For the structure calculations, tunnel models were formed by cutting 7.5 (a–c) and 10.5 (d) units û‹11–20›out of a stack of graphene sheets. The tunnel axis along ‹10–10› is running perpendicular to the paper plane. The front edge is a zig-zag edge, ‹11–20›, running horizontally. For details and a top view, seeSupplementary Fig. S1andSupplementary Methods. Figure 4: Relaxed lowest-energy structures and electron density of tunnels. Structures a – d are the lowest-energy structures after the relaxation. In all lowest-energy structures, the top sheet bends downward. The numbers give the maximum deviation Δ z of the topmost layer from the straight configuration. The bending of surface sheets decreases with increasing number of covering layers ( a – c ) and increases with tunnel width ( a , d ). In density functional theory calculations, no reconfiguration of the electron density is found due to the missing of layers underneath the top sheet ( e ) nor due to bending ( f ). For the structure calculations, tunnel models were formed by cutting 7.5 ( a – c ) and 10.5 ( d ) units û ‹11–20› out of a stack of graphene sheets. The tunnel axis along ‹10–10› is running perpendicular to the paper plane. The front edge is a zig-zag edge, ‹11–20›, running horizontally. For details and a top view, see Supplementary Fig. S1 and Supplementary Methods . Full size image From these calculations, we learn that carbon atoms forming the top of the tunnel will interact with the sheet edges at the side of the tunnel by van der Waals interaction, pulling the layer inward. If two or three layers are bent, roughly two or three times as many bonds have to be stretched, respectively, resulting in less bending as more layers are added. To investigate a possible charge rearrangement, we additionally performed density functional single-point calculations [25] for a whole graphene layer spanning a layer with gap beneath, in either straight ( Fig. 4e ) or bent ( Fig. 4f ) conformations. We find no significant overlap between the density of states of the sheets for either of these conformations. The density-of-states also shows no shift of electrons towards or away from the atoms above the tunnel as compared with the atoms at the sides. Therefore, no essential charge redistribution occurs within the sheet above the tunnel, an effect that is likely to persist if the tunnel is covered by more than one layer of graphene. The findings indicate that the depression in the STM image is indeed caused by a sagging of the graphene sheets on top of a tunnel covered by few-layer graphene. Assuming a spherical shape of the nanoparticle [4] , a tunnel height in the order of magnitude of its width can be inferred. In Fig. 3 , the width can be determined as approximately 12 |û ‹11–20› | shortest distance across the tunnel, corresponding to a height of eight cut layers. The dimensions of the observed tunnel are thus of the same order of size as the tunnels investigated in the models above. Similarly, the measured depressions are of the order of the calculated bending of the cover layers. In our images we find tunnels with different bending, whereas their width is comparable. From the trends in the calculations ( Fig. 4 and Supplementary Table S1 ), we assign this to different number of topping layers and/or differences of the exact tunnel width. Indentations of several Å depth are only observed on wider tunnels or larger irregularly shaped etching “caves”. We also note that interactions between the surface and the tip would pull the top sheet towards the tip [26] , [27] , [28] , therefore counteracting the depression we are observing. As the tip is scanning at rather large distance and we never observe upward bending at our feedback parameters, these forces must be smaller than those within the system. It is interesting to note that a similar appearance in STM, as found for our tunnels and caves, was recently reported for graphene grown over Cu vacancies [28] . Though the interaction with the underlying Cu is necessarily different, resulting in a different depth of the indentation, the general appearance with continuous atomic corrugation, smoothly varying height and no edge enhancement is similar. Triangulation of the tunnel’s depth As a last proof for the existence of tunnels and to estimate if there is a limit, how deep below the surface tunnels can be etched, we performed a triangulation experiment in SEM. The distance between objects in SEM images changes upon tilting due to projection. For objects on the same height level, the distance becomes smaller while their relative position stays the same. Objects on different height level may even change their relative position upon tilting (for geometric details see Supplementary Fig. 2 ). This is observed in Fig. 5 , which shows an SEM image with a trench (marked blue) and a tunnel (marked red) before ( Fig. 5a ) and after tilting the sample by 45° around a horizontal axis ( Fig. 5b ). The tunnel slips past the kink of the trench edge in the upper left corner of Fig. 5 , which immediately shows that the two channels are on different depth levels. From the distance change of the small surface particles (labelled 1–5) relative to the tunnel edge, we calculate a depth of 75 nm below the surface. This is on the order of the theoretical SE escape depth in graphite (100 nm) [29] . The depth at which tunnels can be etched appears to be limited by no other restrictions than the depth of etch pits or the stepped structure of the surface, as tunnels are found at all depth levels, from few layers below the surface (STM) down to the probing limit of SEM. This is not astonishing, as H diffuses readily between graphite sheets. 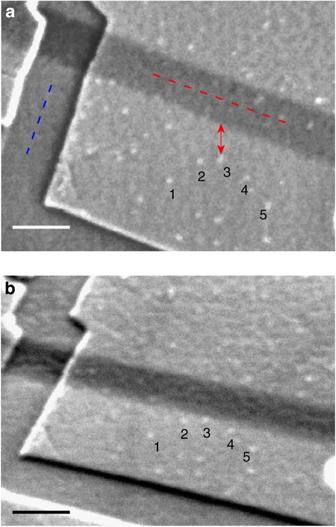Figure 5: Triangulation of the tunnel level. SEM micrographs of a tunnel (red dashes) and a trench (blue dashes), recorded under normal incidence of the electron beam (a) and under an angle of 45° (b; the tilt axis is horizontal). The shift in the relative position between the tunnel and the surface particles (1–5) allows for triangulation of the vertical position of the tunnel with respect to the sample surface (for geometry details seeSupplementary Fig. S2). The length of the red arrow translates into a depth of 75 nm. The lateral tunnel cross-section is 80 nm, which corresponds to 35 nm of covering layers, assuming a circular shape of the tunnel. Scale bars, 100 nm. Figure 5: Triangulation of the tunnel level. SEM micrographs of a tunnel (red dashes) and a trench (blue dashes), recorded under normal incidence of the electron beam ( a ) and under an angle of 45° ( b ; the tilt axis is horizontal). The shift in the relative position between the tunnel and the surface particles (1–5) allows for triangulation of the vertical position of the tunnel with respect to the sample surface (for geometry details see Supplementary Fig. S2 ). The length of the red arrow translates into a depth of 75 nm. The lateral tunnel cross-section is 80 nm, which corresponds to 35 nm of covering layers, assuming a circular shape of the tunnel. Scale bars, 100 nm. Full size image As already reported for etching trenches, we see no indication for tunnels with a direction component perpendicular to the layers, that is, cutting through layers, in our experiments. In general, trenches and tunnels start at step edges and in etch pits (created in a separate preparation step), the particles act on the terminations at the side of the sheets, thus etching parallel to the layers ( Fig. 1b ). From STM images, it is found that the number of layers on top of a tunnel can vary along its length, by one or two layers. Also the etching direction is—on the atomic scale—not strictly straight. We attribute this to a reshaping of the particle on the atomic scale or to local defects in the graphene sheet, which act as nucleation sites for etching and can induce a slight shift of the channel. Etching through whole sheets and thereby forming tunnels in a direction transverse to the layers obviously is highly unfavourable. From our observations, we conclude the following. Although we observe the tunnels with our surface investigation techniques, we stress the fact that the etching mechanism itself is no surface effect, that is, etching does not start from the macroscopic surface of the sample, but we find tunnels that run parallel to the macroscopic surface throughout the probing depth. Because of the diffusion of hydrogen between the layers, etching can occur at all height levels throughout the bulk of the sample, provided that sheet edges are created throughout the bulk and decorated by metal particles. Careful inspection of images in previous publications indicates that tunnel formation may occur also in other systems etched by Ni, Ag and Co [4] , [5] , [6] , [8] , [10] , although it has never been explicitly reported before. This subsurface etching mechanism offers a novel method for fabrication of nanoporous graphite with a high application potential. HOPG is conducting, temperature stable, chemically highly inert and biocompatible. In combination with nanopores, its application in diverse fields is anticipated. As a lithium intercalation material, graphite is widely used as an anode material for Li + -ion batteries. Adjusting the pores in our new material to the ideal size range, the resulting structure allows for fast material transport, that is, the solvent with the ions, to the layer edges. At the same time, the number of edge sites is increased without reducing the storing volume considerably. The material therefore might be a promising candidate for an anode material with improved rate capability [30] , [31] . For life science application, nanoporous graphite could be useful as a drug-eluting, coating material for implants. In contrast to the existing surfaces with nanotubular pores, which provide rough biocompatible implant surfaces for cell growth [32] , [33] , nanoporous graphite could provide the lubricating properties desired for an enhancement of lifetime of sliding contacts in artificial joints [34] supplemented by a depot for drug delivery. Apart from porous material with various tunnel sizes and direction, the pore size could be adjusted to requirements by the use of monodisperse metal particles and even the direction of the channels can be steered by use of magnetic particles [11] . The tunnel walls consist of well-defined hydrogenated sites, which by further chemical substitution, could be functionalized as substance-specific docking sites. Such directed channel growth could provide well-ordered nanochannels for storing or sieving applications, and as scaffolds for molecular architectures. In this respect, the possibility for tunnel formation in other material with graphitic structure, but different electronic properties, should be considered. A promising candidate is BN. When in contact with Ru and exposed to hydrogen at high temperatures, etching occurs by detachment of atoms from the layer edge [35] . Directed etching of nanometre-size tunnels in hexagonal transparent BN [36] would provide a fascinating material for sensing and solar cell applications [37] , [38] . Finally, it was shown by Ci et al. [9] that nano-cut pieces of graphite can be transferred onto insolating surfaces. Similarly, transfer of nanotunnels should be possible, opening—in combination with further lithographic steps—a new route for fabrication and investigation of suspended graphene. In conclusion, we showed that etching HOPG by Ni nanoparticles is not restricted to the surface, resulting in the formation of open trenches. Here we prove, beyond doubt, by high-resolution STM and SEM imaging and triangulation experiments that tunnels are etched underneath the surface. These tunnels are frequently found, and HOPG is perforated by them throughout the probing depth. Quantum chemical models confirmed that the graphene sheets forming the ceiling of tunnels near the surface bend downward due to an attractive interaction with the tunnel walls. No rearrangement of the local electronic structure appears to be associated with this topographic change. The bending increases with increasing width of the tunnel and decreases when the number of covering graphene layers is increased. Our work shows a possible novel preparation method for basic research on graphene and a considerable application potential. Because of the special properties of graphite, this novel form of nanoporous graphite thereby offers a plethora of possibilities for application in various scientific fields. Sample preparation Channels were etched by the two-step preparation method described previously [9] . Freshly peeled HOPG was exposed to air at 650 °C for 1–5 min. Pits with diameter up to several hundred nanometres can be created by this simple oxidation-gasification process. After oxidative etching, we deposited the catalyst by a dip-drawing process. The HOPG piece was immersed into a 0.2 mmol l −1 NiCl 2 /ethanol solution, and then drawn out slowly. After drying in air, the sample was annealed at 500 °C in Ar/H 2 flow (1300, sccm, 15 vol% hydrogen) for 1 h. Then the temperature was immediately increased up to the cutting set-point (900 °C) and held for 1 h. SEM imaging SEM images have been recorded with a Zeiss Ultra Plus SEM using 10 keV primary electrons and the in-lens detector that is expected to be sensitive to SE1 and SE2 secondary electrons [39] . For triangulation, images have been recorded with 30 keV electrons in the high-current mode using the SE2 detector. The sample was tilted relative to the electron beam around an axis, which is parallel to the image’s horizontal axis (details in Supplementary Information ). STM investigations After transfer to the ultra high vacuum chamber, the sample was annealed up to 150 °C for 1 h to remove water and contaminants from air. After cooling to room temperature, it was transferred to our modified Omicron ultra high vacuum variable temperature STM equipped with FEMTO preamplifier. STM tips were electrochemically etched polycrystalline tungsten that was treated by Ar sputtering and annealing in ultra high vacuum. Imaging was performed in constant current mode at room temperature, with the voltage applied to the sample. Linear or polynomial background was substracted from the images, Δ z jumps due to tip reconfigurations have been leveled. No numerical filters have been applied to the images. Theoretical modelling For modelling of the subsurface tunnel, a slab, periodic in the zigzag ‹11–20› and armchair ‹10–10› directions, was modelled. It consists of 5 graphene sheets of 13 periodic units û ‹11–20› along ‹11–20›, and 2 periodic units û ‹10–10› along ‹10–10› direction in AB stacking order (for a detailed geometry see Supplementary Fig. S1 ). Then, a tunnel running along ‹10–10› was created by cutting out the 7.5 central units over the full width for the three inner sheets. The edge of the cut layers runs along ‹10–10›. It corresponds to a straight armchair edge of graphene and was saturated with hydrogen atoms. This results in a tunnel with one whole bottom and top sheet. By adding one or two whole sheets on top, tunnels with two or three topping layers were created. Finally, a wider tunnel was constructed by cutting out the 10.5 central units of the inner 3 layers of a 5-layer stack of width 16 and depth 2 units. Technical details of these calculations are given in the Supplementary Methods . Results for the bending of additional geometries are listed in Supplementary Table 1 . Programs used For STM image processing, the programme gwyddion was used. The images in Fig. 1 are produced by POV-ray ray tracing software. Viewgraphs have been prepared by OriginPro. How to cite this article : Lukas, M et al. Catalytic subsurface etching of nanoscale channels in graphite. Nat. Commun. 4:1379 doi: 10.1038/ncomms2399 (2013).